Systematic identification of genes with a cancer-testis expression pattern in 19 cancer types Cancer-testis ( CT ) genes represent the similarity between the processes of spermatogenesis and tumorigenesis. It is possible that their selective expression pattern can help identify driver genes in cancer. In this study, we integrate transcriptomics data from multiple databases and systematically identify 876 new CT genes in 19 cancer types. We explore their relationship with testis-specific regulatory elements. We propose that extremely highly expressed CT genes (EECTGs) are potential drivers activated through epigenetic mechanisms. We find mutually exclusive associations between EECTGs and somatic mutations in mutated genes, such as PIK3CA in breast cancer. We also provide evidence that promoter demethylation and close non-coding RNAs (namely, CT-ncRNAs) may be two mechanisms to reactivate EECTG gene expression. We show that the meiosis-related EECTG ( MEIOB ) and its nearby CT-ncRNA have a role in tumorigenesis in lung adenocarcinoma. Our findings provide methods for identifying epigenetic-driver genes of cancer, which could serve as targets of future cancer therapies. Over the past decade, genome-wide analyses via exome sequencing have become routine in cancer research. Large cooperative projects such as The Cancer Genome Atlas (TCGA), as well as other independent studies, have identified hundreds of genes that may promote tumorigenesis when altered by intragenic mutations [1] , [2] , [3] . These findings dramatically expand the range of targetable alterations and ultimately advance personalized therapy. However, individuals with the same tumour type are highly heterogeneous and contain diverse genomic alterations [4] , [5] . Studies suggest that only a few mutations in these mutation-driver ( mut-driver ) genes are sufficient to trigger cancer [1] , [3] , [6] . The remaining mutations are passengers that confer no selective growth advantage. The majority of somatic point mutations present with low population frequencies [1] , [2] , [7] , [8] , [9] , [10] , [11] , with only a handful of mutations observed in >5% of patients. In 12 major cancers investigated in the TCGA project [1] , only 10 significantly mutated genes (SMGs) contain point mutations in >5% of samples. Thus, few cancers can be completely explained by known driver mutations. Epigenetic alterations, which lead to aberrant expression patterns, are now acknowledged as a universal feature of tumorigenesis. In turn, aberrant expression patterns are an important characteristic of epigenetic-drivers (epi-drivers) [3] . In the present study, we observed a group of genes in which expression was restricted to germ cells and often reactivated and aberrantly expressed in tumour cells. These gene products were named cancer/testis (CT) antigens in initial studies due to their immunogenicity [12] , [13] . The existence of these genes reflects the similarities between the processes of gametogenesis and tumorigenesis. Study of these genes provides valuable understanding of tumorigenesis [12] . The reactivation of these genes in cancer samples makes them oncogene candidates, and their restricted expression profile in normal tissues makes them potential targets for therapy. CT antigens were first identified by autologous typing [14] . The rapid development of PCR and microarray technology accelerated the identification processes based on the expression patterns of these genes [15] , [16] , [17] , [18] . To date, more than 200 genes have been recorded as CT genes in public databases [19] . Although great success has been achieved [17] , [18] , [19] , research on CT genes still faces many challenges. First, most studies have examined expression patterns in only a small number of samples [18] . The lack of transcriptomics data from a large number of normal tissue samples of multiple types as well as high-quality cancer samples has made it difficult to systematically and comprehensively evaluate these genes. Second, hundreds of CT genes are listed in databases; how they are reactivated and whether these reactivated testis proteins support tumorigenic features remains to be studied thoroughly. Some genes, such as LIN28B , have been reported to act as oncogenes in specific cancers [20] , [21] , [22] , [23] , [24] . However, the CT expression patterns of these genes have been ignored. Third, these genes have been pursued as targets for anticancer vaccines; however, researchers may have ignored the possibility that these genes could be useful targets of molecular-targeted therapy. For example, use of the CT antigen BRDT as a contraceptive target has been proposed due to its high efficacy and the minimal side effects associated with this therapeutic strategy [25] . Recently, databases such as The Genotype-Tissue Expression (GTEx) [26] , [27] , [28] and TCGA [29] have provided a great deal of transcriptomic data from normal and tumour tissues and provided opportunities to identify CT genes and to explore the similarities and differences between spermatogenesis and tumorigenesis. In this study, we performed a comprehensive, multiplatform analysis on large, independent and publically available databases (GTEx, HPM, TCGA, The Encyclopedia of DNA Elements (ENCODE), The Functional Annotation of The Mammalian Genome (FANTOM) and so on) and our data (NJMU-seq) to systematically identify and describe CT genes. We further defined extremely highly expressed CT genes (EECTGs) to indicate potential epi-driver genes and explore the correlation between these genes and mutations, promoter methylation levels and nearby non-coding RNAs (ncRNAs). After subsequent validation, we demonstrated that a meiosis-related EECTG ( MEIOB ) and its companion testis-specific ncRNA (TS-ncRNA; LINC00254 ) play crucial roles in carcinogenesis in lung adenocarcinoma (LUAD). Testis-specific genes and their enriched characteristics To identify CT genes at a genome-wide scale, we first defined testis-specific genes (TSGs) and classified all human genes into six categories based on expression patterns ( Supplementary Fig. 1 ). We used three independent transcriptomic data sets from normal tissues ( Supplementary Data 1 ) and defined TSGs including TS-ncRNAs. We found that 8,565 genes (17.12% of 50,016 GENCODE genes, Version 19) exhibited testis-specific expression patterns ( Fig. 1a , Supplementary Data 2 ). Among them, 1,336 genes (2.67%) were protein-coding genes with higher confidence (C1) and were considered as candidate CT genes for further analysis. Among the genes not expressed predominantly in testis in the GTEx database (C6), some were classified as testis-specific transcripts (C6a, 8.28%); for these genes, at least one transcript was expressed exclusively in the testis. It is also worth noting that thousands of ncRNAs (10.08%, C2 and C4) showed testis-specific expression ( Fig. 1a ). Most of these non-coding genes (94.1%) were annotated as long ncRNAs (lncRNAs), pseudogenes or antisense RNAs based on the GENCODE v19 reference. Most of these genes (98.4%) did not share exons with protein-coding genes. 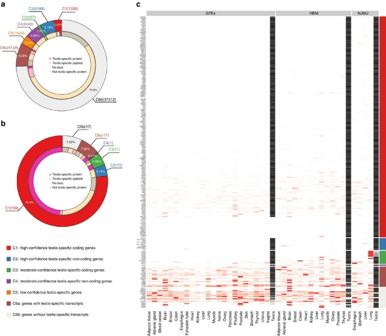Figure 1: Classification of all genes and knownCTgenes. (a) All 50,016 genes were classified into six groups according to their mRNA expression patterns and classified into three groups according to their protein expression patterns. The pie chart displays the mRNA expression classification in the outer circle and the protein expression classification in the inner circle. (b) Pie chart summary of the classification of knownCTgenes. mRNA expression and protein abundance of knownCTgenes. The genes in theyaxis were ranked by the SPM values from the GTEx database in descending order. The expression of each gene was rescaled to the interval [0, 1]. The depth of colour indicates the expression level. Black indicates testis and red indicates other normal tissues. The colour of each category corresponds with the colours ina,b. Genes were classified into the following six categories based on specificity measure (SPM) values: (C1) high-confidence testis-specific coding genes: GENCODE-annotated protein-coding genes (v19) with (a) SPMGTEx>0.9, SPMHBM>0.9 and SPMNJMU>0.9; or (b) Known CT and SPMGTEx=0, SPMHBM>0.9, SPMNJMU>0.9 and gene copies with identical sequences; (C2) high-confidence testis-specific non-coding genes: GENCODE-annotated non-coding genes (v19) with SPMGTEx>0.9, SPMHBM>0.9 and SPMNJMU>0.9; (C3) moderate-confidence testis-specific coding genes: GENCODE-annotated protein-coding genes (v19) with SPMGTEx>0.9 and either SPMHBM>0.9 or SPMNJMU>0.9; (C4) moderate-confidence testis-specific non-coding genes: GENCODE-annotated non-coding genes (v19) with SPMGTEx>0.9 and either SPMHBM>0.9 or SPMNJMU>0.9; (C5) low-confidence testis-specific genes: genes with SPMGTEx>0.9 but SPMHBM≤0.9 and SPMNJMU≤0.9; (C6) non-gene-level testis-specific gene: genes with SPMGTEx≤0.9.G6genes were then classified into the following two sub-groups using transcript abundance data from GTEx; (C6a) genes with testis-specific transcripts: C6 with SPMGTEx transcript>0.9; (C6b) genes without testis-specific transcripts: C6 with SPMGTEx transcript≤0.9. (c) Complete expression patterns of known CT genes in the GTEx, HBM and NJMU studies. Figure 1: Classification of all genes and known CT genes. ( a ) All 50,016 genes were classified into six groups according to their mRNA expression patterns and classified into three groups according to their protein expression patterns. The pie chart displays the mRNA expression classification in the outer circle and the protein expression classification in the inner circle. ( b ) Pie chart summary of the classification of known CT genes. mRNA expression and protein abundance of known CT genes. The genes in the y axis were ranked by the SPM values from the GTEx database in descending order. The expression of each gene was rescaled to the interval [0, 1]. The depth of colour indicates the expression level. Black indicates testis and red indicates other normal tissues. The colour of each category corresponds with the colours in a , b . Genes were classified into the following six categories based on specificity measure (SPM) values: (C1) high-confidence testis-specific coding genes: GENCODE-annotated protein-coding genes (v19) with ( a ) SPM GTEx >0.9, SPM HBM >0.9 and SPM NJMU >0.9; or ( b ) Known CT and SPM GTEx =0, SPM HBM >0.9, SPM NJMU >0.9 and gene copies with identical sequences; (C2) high-confidence testis-specific non-coding genes: GENCODE-annotated non-coding genes (v19) with SPM GTEx >0.9, SPM HBM >0.9 and SPM NJMU >0.9; (C3) moderate-confidence testis-specific coding genes: GENCODE-annotated protein-coding genes (v19) with SPM GTEx >0.9 and either SPM HBM >0.9 or SPM NJMU >0.9; (C4) moderate-confidence testis-specific non-coding genes: GENCODE-annotated non-coding genes (v19) with SPM GTEx >0.9 and either SPM HBM >0.9 or SPM NJMU >0.9; (C5) low-confidence testis-specific genes: genes with SPM GTEx >0.9 but SPM HBM ≤0.9 and SPM NJMU ≤0.9; (C6) non-gene-level testis-specific gene: genes with SPM GTEx ≤0.9. G6 genes were then classified into the following two sub-groups using transcript abundance data from GTEx; ( C6a ) genes with testis-specific transcripts: C6 with SPM GTEx transcript >0.9; ( C6b ) genes without testis-specific transcripts: C6 with SPM GTEx transcript ≤0.9. ( c ) Complete expression patterns of known CT genes in the GTEx, HBM and NJMU studies. Full size image Using this classification, which included testis-specific transcripts, a majority (226, 92.98%) of the 243 known CT genes [19] satisfied our criteria in the GTEx project (C1–C6a, Fig. 1b,c ). However, seventeen known CT genes (C6b) were widely expressed in more than one tissue ( Fig. 1b,c ). Due to limitations in protein quantification technology, most previous studies defined TSGs at the mRNA level. The correlation between mRNA and protein expression is a matter of scientific debate, and studies have suggested that the process of translation from mRNA to protein is complicated. In this study, we used human proteomic data from 16 different normal adult tissues [30] ( Supplementary Data 1 ) to define testis-specific proteins (TSPs). Peptides mapped to multiple proteins may bias the evaluation of testis-specific expression. Some classical CT genes, such as genes from MAGE family, have similar sequences and shared peptides, making it challenging to define TSPs. To resolve this issue, we examined expression at both the protein and the peptide level in this analysis (Methods section). Of the 15,297 proteins annotated in the GENCODE databases, 1,218 proved to be TSPs; 418 were consistent with the TSGs from group C1 ( Fig. 1a ). The relatively small proteomic data sample size may have contributed to this inconsistency, especially for rarely expressed genes. Half of the TSGs in C1 were not expressed as protein in testis, indicating that there may be differences between mRNA estimations and protein abundance (for example, in quantification sensitivities or expression cutoffs). We cannot exclude the possibility that some TSGs may not be translated in the testis even though their mRNA level was high. We also observed TSPs without testis-specific mRNA expression. The occurrence of these genes may be due to the conservative alignment strategy of RNA-sequencing (RNA-Seq) data on genes with similar sequence ( CXorf49 and CXorf49B ) or the presence of transcripts with different expression patterns (both testis-specific transcripts and non-testis-specific transcripts). Compared with the coding genes in C6b (non-TSGs), TSPs were significantly enriched as C1 genes (enrichment ratio (ER)=23.47, Fisher’s exact test P =6.01 × 10 −283 ). We further examined whether regulatory elements (promoters, enhancers, ncRNAs or methylation sites) were involved in TSG expression patterns in the testis. By integrating data from Cap Analysis of Gene Expression analyses released by the FANTOM project and data from Reduced Representation Bisulfite Sequencing analyses released by the ENCODE project, we found that testis-specific promoters and demethylation sites were frequently located proximally upstream (−100 to 1 kb) of C1 genes (ER promoter =10.10, Fisher’s exact test P promoter =6.42 × 10 −253 ; ER methylation =5.37, Fisher’s exact test P methylation =6.57 × 10 −12 , Fig. 2 ). Furthermore, testis-specific ncRNAs were typically located 100 kb upstream or downstream of C1 genes ( Fig. 2 ). However, enrichment of testis-specific enhancers was not observed for C1 genes ( Fig. 2 ). 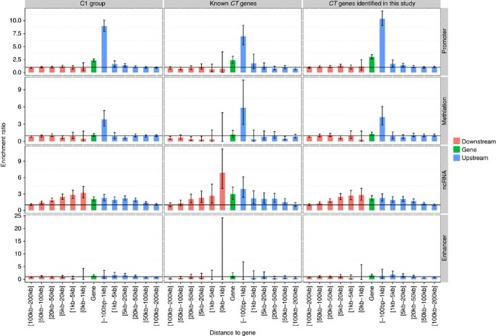Figure 2: Enrichment analysis of testis-specific regulatory elements (TSREs). Enrichment analysis was used to evaluate the relationship betweenTSREsandCTgenes. Four types of regulatory elements (promoters, methylation sites, non-coding RNAs and enhancers) were included in the analysis. The error bar represents the ER confidence interval. Figure 2: Enrichment analysis of testis-specific regulatory elements (TSREs). Enrichment analysis was used to evaluate the relationship between TSREs and CT genes. Four types of regulatory elements (promoters, methylation sites, non-coding RNAs and enhancers) were included in the analysis. The error bar represents the ER confidence interval. Full size image CT genes and their reactivation in cancers The TCGA project provides publically available expression profiles from thousands of cancer patients. Using these data, we distinguished CT genes from TSGs with higher confidence ( C1 genes). We included 19 cancer types in which expression abundance was observed from mRNA sequencing in our analysis ( Supplementary Data 1 ). As listed in Supplementary Data 3 , 1,019 (77%) of the 1,336 C1 genes that were expressed in at least 1% of the samples (>5 normalized read counts) of any cancer type were CT genes for the particular cancer. We observed a similar enrichment pattern for regulatory elements for genes defined in our study as C1 genes and known CT genes ( Fig. 2 ). Previous studies have demonstrated that known CT genes are aberrantly activated in up to 40% of various cancer types [17] . Because of our large study sample size and advances in RNA sequencing technology [31] , we found that many CT genes (37.2–59.1%) were expressed in more than 40% of samples for each cancer type. For these genes, expression in most of the samples was relatively low; these genes may not play an important role in tumorigenesis. Because adjacent cancer tissues usually do not express CT genes, it was challenging to determine activated samples individually. Here we considered samples with extremely high expression (EE; Methods section) as samples activated for the CT gene. CT genes identified in at least 1% of EE samples were defined as EECTGs for a particular cancer. In total, 891 of the 1,019 identified CT genes passed these criteria for at least one cancer type ( Supplementary Data 3 ); 300 EECTPs (extremely highly expressed CT proteins: EECTGs with TSP expression) were selected for further analysis. We found that C1 genes were approximately twice as likely to display this EE pattern in cancer samples compared with non-TSGs (ER=2.05, Fisher’s exact test P =2.21 × 10 −22 , Fig. 3a ). This finding indicates that TSGs were more likely to display this EE pattern in tumour tissues. Similar to the mutation spectrum observed in cancer [1] , [3] , the maximum EE frequency was <7% in each cancer type. Genes with EE patterns were very rare (median: 0–2) in each cancer sample. Some cancer types, such as pancreatic ductal adenocarcinoma, kidney renal papillary cell carcinoma, lower grade glioma and glioblastoma, presented with an average of 0 EECTPs and were considered to be ‘CT poor cancers’ ( Fig. 3b ). We also measured CT gene expression in 24 LUAD samples by RNA sequencing and validated 19 EECTPs (7 novel, Supplementary Fig. 2 ). 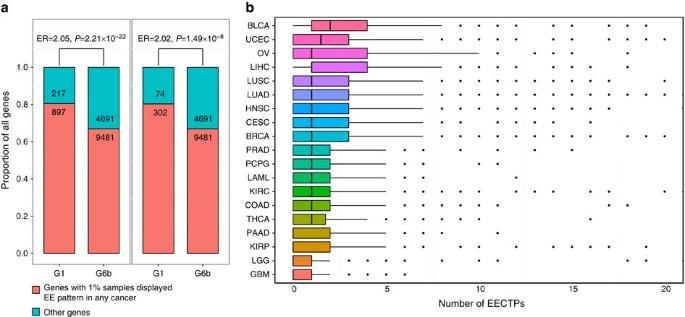Figure 3: General description of EECTPs in 19 cancer types. (a) Enrichment analysis suggests that EE patterns were more likely to emerge in TSGs and TSPs, Fisher's exact test was applied to evaluate the enrichment ratio. (b) Number of activated EECTPs in 19 cancer types. The box plot displays the first and third quartiles (top and bottom of the boxes), the median (band inside the boxes), and the lowest and highest point within 1.5 times the interquartile range of the lower and higher quartile (whiskers). Figure 3: General description of EECTPs in 19 cancer types. ( a ) Enrichment analysis suggests that EE patterns were more likely to emerge in TSGs and TSPs, Fisher's exact test was applied to evaluate the enrichment ratio. ( b ) Number of activated EECTPs in 19 cancer types. The box plot displays the first and third quartiles (top and bottom of the boxes), the median (band inside the boxes), and the lowest and highest point within 1.5 times the interquartile range of the lower and higher quartile (whiskers). Full size image For a more global analysis of TSGs and EECTPs, we performed a gene ontology analysis using the DAVID platform [32] . The top 10 clusters are shown in Supplementary Data 4 . Genes involved in reproduction-related process were consistently enriched as TSGs and EECTPs. As the function of most CT genes in the development of cancer remained unknown, the information we obtained from the gene ontology term analysis was limited. Exclusive patterns of activation of EECTPs and mutations SMGs are commonly thought to be the major source of mut-driver genes [1] , [3] . Our aim in this study was to explore the relationship between the expression of EECTPs and the mutation of SMGs. Eight types of major cancers within the TCGA were selected for the analysis if more than 100 platform-overlapping samples were available. We used the proportion of somatic mutation numbers in SMGs and in all genes (the SMG mutation ratio) to represent the degree of samples driven by SMG mutation. We used the number of activated EECTPs to represent the proportion of samples driven by EECTPs. Interestingly, we found that the number of activated EECTPs was inversely associated with the SMG mutation ratio after adjusting for cancer type ( β =−4.58, linear regression P =8.28 × 10 −5 , Supplementary Fig. 3a ). However, no significant association between the number of activated EECTPs and the mutation ratio of EECTPs was observed ( Supplementary Fig. 3b ). In many cancers, we noticed that the number of activated EECTPs was significantly higher in TP53 mutated samples (adjusted by false discovery rate (FDR), P <0.05, Supplementary Fig. 4a ). Because TP53 is a gatekeeper for genome instability, we excluded TP53 gene mutations when calculating the SMG mutation ratio, which resulted in a more obvious negative correlation ( β =−5.75, linear regression P =6.87 × 10 −7 , Supplementary Fig. 3c ). We further evaluated the correlation between the mutation pattern of each SMG and the activation of each EECTP. Because the frequency of mutations and EECTPs’ activation were both low, we performed this analysis only in breast cancer (BRCA), which had the largest sample size. Eight SMGs were significantly associated with the activation of EECTPs ( Supplementary Fig. 4b ). However, only PIK3CA was consistently associated with the activation of EECTPs in multiple molecular subtypes ( Supplementary Fig. 4c ). As PIK3CA is a well-known BRCA oncogene, we further explored the correlation between each EECTP and mutations in PIK3CA ( Supplementary Data 5 ). This analysis revealed that the relationship between the activation of multiple EECTPs was mutually exclusive with mutations in PIK3CA (FDR adjusted, P <0.05, Fig. 4a ); these findings included MEIOB . CT gene expression was enriched in basal-like BRCA samples, which have a lower PIK3CA mutation frequency ( Fig. 4b ). This suggests that the activation of EECTPs may also be related to molecular subtypes of BRCA. A recent study identified multiple mut-driver genes in a handful of samples and clearly defined mutually exclusive driver genes for patients with papillary thyroid carcinoma. This provided us with an opportunity to study the correlation between EECTPs and mut-driver genes. As expected, the total of number of activated EECTPs was significantly higher in patients without clear driver alterations ( Fig. 4c ). Moreover, we identified four EECTPs prone to activation in patients without driver mutations. We observed that the activation of MEIOB was restricted in patients without driver mutations or fusions. Almost all MEIOB -activated patients had driving arm-level copy number alterations. This evidence suggests that the activation of EECTPs may complement alterations in known driver genes. 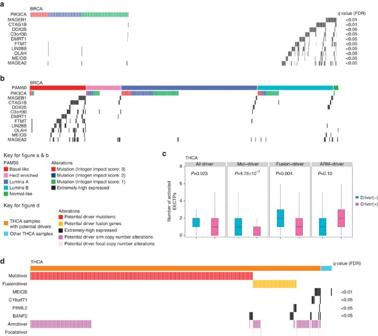Figure 4: The association between the activation pattern of EECTPs and the alterations of the driver genes in patients with BRCA and papillary thyroid carcinoma. (a) Mutually exclusive pattern of EECTP activation andPIK3CAmutation in breast cancer. (b) Mutually exclusive pattern of EECTP activation andPIK3CAmutation in different PAM50 subtypes. (c) The total of number of activated EECTPs is significantly higher in papillary thyroid carcinoma patients without clear driver alterations (mutations and fusions). The box plot displays the first and third quartiles (top and bottom of the boxes), the median (band inside the boxes), and the lowest and highest point within 1.5 times the interquartile range of the lower and higher quartile (whiskers). (d) The activation ofMEIOBis restricted in papillary thyroid carcinoma patients without driver mutations or fusions but co-occur with arm copy number drivers. Figure 4: The association between the activation pattern of EECTPs and the alterations of the driver genes in patients with BRCA and papillary thyroid carcinoma. ( a ) Mutually exclusive pattern of EECTP activation and PIK3CA mutation in breast cancer. ( b ) Mutually exclusive pattern of EECTP activation and PIK3CA mutation in different PAM50 subtypes. ( c ) The total of number of activated EECTPs is significantly higher in papillary thyroid carcinoma patients without clear driver alterations (mutations and fusions). The box plot displays the first and third quartiles (top and bottom of the boxes), the median (band inside the boxes), and the lowest and highest point within 1.5 times the interquartile range of the lower and higher quartile (whiskers). ( d ) The activation of MEIOB is restricted in papillary thyroid carcinoma patients without driver mutations or fusions but co-occur with arm copy number drivers. Full size image EECTPs may be regulated by promoter methylation levels By integrating DNA methylation data from TCGA, we further explored the relationship between the activation of EECTPs and the methylation level of their promoters. Seven cancer types were selected from the major TCGA cancers with more than 100 platform-overlapped samples and were included in our analysis. The average promoter methylation levels of EECTPs were negatively associated with activated EECTP numbers ( β =−30.97, linear regression P =9.68 × 10 −97 , Fig. 5 ) after adjusting for cancer type. When the average promoter methylation level of all genes was considered to exclude the influence of genome-wide hypomethylation, the negative association remained ( β =−56.38, linear regression P =1.68 × 10 −52 ). 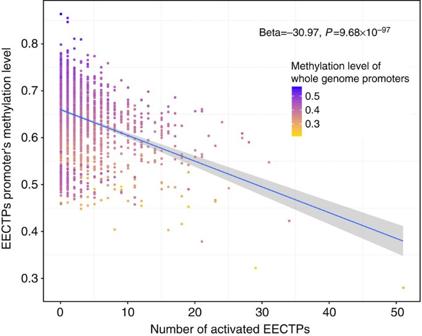Figure 5: Negative correlation between the average promoter methylation level of EECTPs and the number of activated EECTPs. The depth of colour indicates the genome-wide promoter methylation level. The blue line is the best-fit linear regression and the shaded area indicates the confidence interval. Figure 5: Negative correlation between the average promoter methylation level of EECTPs and the number of activated EECTPs. The depth of colour indicates the genome-wide promoter methylation level. The blue line is the best-fit linear regression and the shaded area indicates the confidence interval. Full size image We further compared methylation levels between EE and non-EE samples for each EECTP in the corresponding cancer type. For LUAD, BRCA and head and neck squamous cell carcinoma, more than half of EECTPs exhibited differential methylation levels between EE and non-EE samples ( Supplementary Data 6 ). We validated seven EECTPs in our LUAD samples. Of these, two genes ( TSPY1 and RBMY1A1 ) were located on the Y chromosome; promoter methylation information was not included in the Illumina 450 k methylation array. Two genes proved to be significantly demethylated in EE samples ( RHOXF1 and VCX3B , Supplementary Fig. 5 ), suggesting that these genes may be reactivated through aberrant promoter methylation. The remaining genes ( LIN28B , MEIOB and SPATA22 ) may be activated by an alternative mechanism in LUAD. CT ncRNA As noted above, we found thousands of non-coding genes with testis-specific expression (TS-ncRNAs; C2 and C4). To better understand the expression patterns of TS-ncRNAs in cancer samples, we used two data sets from recently published papers. One study provided us with expression abundance data for 1,791 differentially expressed ncRNAs in TCGA [33] . We found that 239 of these ncRNAs were TS-ncRNAs (namely, CT-ncRNAs; Supplementary Data 7 ). Another study performed de novo assembly of ncRNAs from the TCGA data and released expression abundance data for cancer/lineage-associated ncRNAs [34] . Based on these differentially expressed ncRNAs, we successfully annotated 967 ncRNAs using transcripts from GENCODE v19; annotations were performed using coordinates that overlapped with the reference ncRNAs ( Supplementary Methods ). Of these ncRNAs, 173 were CT-ncRNAs ( Supplementary Data 7 ). We further explored whether the expression of CT-coding genes was influenced by CT-ncRNAs and found 174 and 258 cancer-specific CT-coding gene/CT-ncRNA pairs (where the distance between the CT-coding gene and CT-ncRNA was <100 kb) from the two studies. Many pairs displayed significant correlation ( P FDR <0.05), suggesting that close relationships exist between CT-coding genes and CT-ncRNAs ( Supplementary Data 8 ). Among these CT-coding gene/CT-ncRNA pairs, some genes have been reported to participate in cancer or spermatogenesis. For example, DEPDC1 was reported to contribute to bladder cancer oncogenesis by interfering with the transcriptional repressor ZNF224 (ref. 35 ). PWRN1 was reported to be a part of the IC-SNURF-SNRPN transcription unit, which may be involved in the process of spermatogenesis [36] . Without the expression data for all of ncRNA transcripts in the TCGA, we cannot evaluate focally activated ncRNAs comprehensively. Using our LUAD samples, we identified a TS-ncRNA ( LINC00577 ) that was correlated with the expression of LIN28B (Spearman’s rank correlation coefficient=0.42, P =0.04). This finding suggests that CT genes may be activated by nearby TS-ncRNAs. MEIOB is a meiosis-related epi-driver candidate in LUAD Of the seven EECTPs mentioned above, we observed that MEIOB and SPATA22 were recently reported to be essential factors acting during meiotic recombination. MEIOB exhibits 3′–5′ exonuclease activity and localizes to meiotic chromatin by forming a complex with SPATA22. Thus, MEIOB is essential for meiotic recombination. SPATA22 may modulate the nuclease activity and substrate specificity of MEIOB [37] . First, we explored the co-expression patterns of these two genes in testis and tumour tissues. We found that the expression of MEIOB and SPATA22 was significantly correlated in 14 GTEx normal testis tissues ( Fig. 6a ). Most interestingly, the EE patterns of these two genes were mutually exclusive in patients with LUAD ( Fig. 6b ). We also observed similar MEIOB and SPATA22 activation in other tumour types ( Supplementary Fig. 6 ). 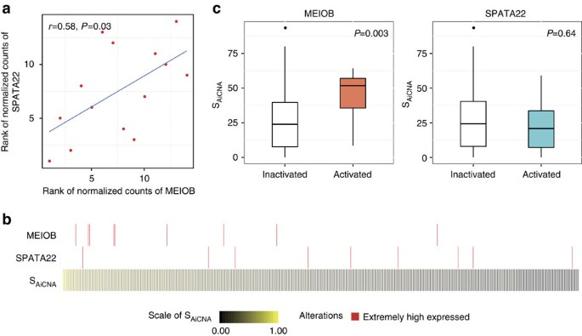Figure 6:MEIOBandSPATA22co-expression patterns in testis and tumour samples and the association between MEIOB activation and SAi. (a)MEIOBandSPATA22are co-expressed in testis. (b)MEIOBandSPATA22are exclusively activated in LUAD samples. (c) Activation ofMEIOBis associated with higher SAi. The box plot displays the first and third quartiles (top and bottom of the boxes), the median (band inside the boxes), and the lowest and highest point within 1.5 times the interquartile range of the lower and higher quartile (whiskers). Figure 6: MEIOB and SPATA22 co-expression patterns in testis and tumour samples and the association between MEIOB activation and S Ai . ( a ) MEIOB and SPATA22 are co-expressed in testis. ( b ) MEIOB and SPATA22 are exclusively activated in LUAD samples. ( c ) Activation of MEIOB is associated with higher S Ai . The box plot displays the first and third quartiles (top and bottom of the boxes), the median (band inside the boxes), and the lowest and highest point within 1.5 times the interquartile range of the lower and higher quartile (whiskers). Full size image In addition, the expression of MEIOB was positively correlated with the genome-wide burden of focal copy number aberrations (CNAs) among samples from 10 cancer types with MEIOB and SPATA22 activation (Spearman’s rank correlation coefficient=0.12, P =8.30 × 10 −14 ). The correlation was significant ( P <0.05) in LUAD samples and samples from other cancer types (bladder urothelial carcinoma: P =0.008; BRCA: P =0.02; thyroid carcinoma: P =0.05; uterine corpus endometrial carcinoma: P =0.01). To unravel the potential aneuploidy formation mechanism in which MEIOB may be involved, we recalled allele-specific copy number alternations and calculated the score of allele-imbalanced events using the method described previously [38] . Similar to a previous report concerning HORMAD1 (ref. 38 ), we found that the activation of MEIOB significantly increased the signal of allele-imbalanced alternations (the score of allele-imbalanced CNAs and copy-neutral loss of heterozygosity (CnLOH)) in LUAD samples ( Fig. 6c ). To prove that MEIOB plays a critical role during the development of cancer, we designed a series of in vitro experiments. Expression pattern of MEIOB in normal and LUAD tissues were displayed in Fig. 7a,b . The overexpression of MEIOB in A549 cells resulted in increased cell viability and malignant phenotypes. Deletion of MEIOB inhibited clonogenicity as well as cell growth, invasion and migration ( Fig. 7c,d , Supplementary Fig. 7 ). We further demonstrated that the overexpression of MEIOB in A549 cell lines resulted in a significantly reduced population of S phase cells and an increased population of G2 phase cells. Deletion of MEIOB led to opposite results. In addition to coding genes, we identified a TS-ncRNA ( LINC00254 ) near MEIOB . LINC00254 is located 6 kb upstream of MEIOB . It is a testis-specific expressed transcript ( Fig. 7a ) and is expressed in samples without MEIOB activation ( Fig. 7b ); however, LINC00254 was not expressed in any of the LUAD cell lines tested ( Supplementary Fig. 8a,b ). In the A549 cell line, the stable overexpression of LINC00254 downregulated MEIOB and produced results similar to those seen in the MEIOB knockout ( Fig. 7e , Supplementary Figs 7 and 8c ). We further performed cell cycle assay in MEIOB overexpressing and knockout A549 cell lines. We observed that the overexpression of MEIOB in A549 cell lines resulted in significantly reduced population of S phase cells and increased population of G2 phase cells ( Fig. 7f ). On the contrary, the deletion of MEIOB led to opposite results ( Fig. 7g ). These results suggest that MEIOB may participate in the process of tumorigenesis by damaging genome stability. LINC00254 may act as a natural inhibitor of MEIOB . 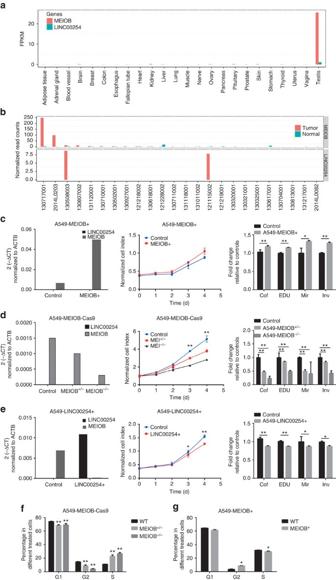Figure 7:MEIOB/LINC00254drive lung cancer cell growth, migration and invasionin vitro. (a) Expression ofMEIOB/LINC00254in the GTEx data sets. (b) Expression ofMEIOB/LINC00254in our 24 tumour/normal paired samples. (c) Overexpression ofMEIOBeffects A549 vitality. (d) Knockout ofMEIOBeffects A549 vitality. (e) Overexpression ofLINC00254effects A549 vitality. Relative expression ofLINC00254andMEIOB(left) and a growth curve (middle) of different treated A549 cells. The fold change is relative to the control of colony formation; EdU staining, migration and invasion are shown together (right). (f) Cell cycle distribution in the A549 control andMEIOBknockout cells. (g) Cell cycle distribution in the A549 control andMEIOBoverexpressing cells. Error bars represent s.e.m,n=5. *P<0.05 compared with the vector control. **P<0.001 compared with the vector control. All of the experiments were repeated three times. Figure 7: MEIOB/LINC00254 drive lung cancer cell growth, migration and invasion in vitro . ( a ) Expression of MEIOB / LINC00254 in the GTEx data sets. ( b ) Expression of MEIOB / LINC00254 in our 24 tumour/normal paired samples. ( c ) Overexpression of MEIOB effects A549 vitality. ( d ) Knockout of MEIOB effects A549 vitality. ( e ) Overexpression of LINC00254 effects A549 vitality. Relative expression of LINC00254 and MEIOB (left) and a growth curve (middle) of different treated A549 cells. The fold change is relative to the control of colony formation; EdU staining, migration and invasion are shown together (right). ( f ) Cell cycle distribution in the A549 control and MEIOB knockout cells. ( g ) Cell cycle distribution in the A549 control and MEIOB overexpressing cells. Error bars represent s.e.m, n =5. * P <0.05 compared with the vector control. ** P <0.001 compared with the vector control. All of the experiments were repeated three times. Full size image It has long been acknowledged that the processes of germ cell development and tumour development share important similarities, including immortalization, the induction of meiosis, invasion and migration [12] . The products of these gamete-specific genes may be deleterious for the orderly requirements of normal somatic cells and highly advantageous in cancer cells. Thus, the systematic evaluation of the transcriptomes of germ cells and tumour samples may help us identify key elements involved in both gametogenesis and tumorigenesis and understand their differences. In the present study, we integrated multiple independent transcriptome databases containing both normal and tumour samples and systematically explored the molecular landscape of CT genes. Detailed information concerning the CT genes mentioned in this article is freely accessible through our search engine (CTatlas: http://reprod.njmu.edu.cn/ctatlas/ ). CT genes were first observed and considered to be candidate targets for immunotherapy due to their immunogenicity. Since then, immunogenicity has been regarded as one of the most important characteristics of CT genes. However, 18 of the 23 phase II/III clinical trials that tested 17 distinct therapeutic anticancer vaccines failed to achieve their primary objectives; this included a trial for the vaccine targeting MAGEA3 in non-small cell lung cancer [39] , [40] , [41] . Frustrations concerning clinical experiments indicate the great challenges present in the development of immunotherapy without the sufficient identification of the expression patterns of CT genes. Further characterization of the role of epi-drivers and the reactivation mechanism of CT genes would greatly benefit the development of therapeutic strategies. With the development of cancer genomics, molecular-targeted therapies are increasingly used as an alternative to chemotherapy [42] , [43] . The development of targeted therapies requires the identification of targets that play a key role in cancer cell growth and survival. Because CT genes are normally expressed exclusively in the testis but frequently turned on in many types of tumours, there is a significant possibility that CT genes are involved in the process of tumorigenesis. CT genes are therefore considered to be epi-driver candidates, which have been described as one of the major sources of ‘dark matter’ in cancer. MAGEA3 serves as an example; although a clinical trial of an immunotherapy targeting MAGEA3 was suspended because it failed to improve the survival of patients with non-small cell lung cancer, MAGEA3 was recently reported to be necessary for cancer cell viability and sufficient to drive the tumorigenic properties of non-cancerous cells [44] . Therefore, efforts to inhibit MAGEA3 should not be halted. Rather, failed approaches should be replaced with a more suitable individualized therapy plan. In our study, we considered genes that were extremely highly expressed in more than 1% of the samples as potential candidates for epi-drivers. Consistent with previous studies [44] , MAGEA3 was defined as an EECTP in multiple cancer types (BRCA, colon adenocarcinoma, glioblastoma and so on, Supplementary Data 3 ). Thus, cases with extremely high MAGEA3 expression in our study may be ideal candidates for a future therapy targeting MAGEA3 and may benefit from such treatment. Meiosis in gametogenesis and aneuploidy in tumorigenesis share similar characteristics and mechanisms [12] . The induction of DNA double-strand breaks, which increases genome diversity and is essential for proper chromosome segregation at the first meiotic division [45] , is an important process during meiotic recombination. Mitosis inhibits this process; mitosis can lead to telomere fusions that produce dicentric chromosomes and aneuploidy, especially in the presence of exogenous genotoxic stress [46] . A recent study identified a CT gene involved in the promotion of nonconservative recombination in meiosis as a novel driver of an allelic imbalance phenotype in triple-negative BRCA [38] . In this study, we also observed the activation of a CT gene, MEIOB . MEIOB exhibits 3′–5′ exonuclease activity during meiotic recombination and is essential for meiosis [37] . This activity may contribute to the genome instability observed in LUAD patients. The co-factor for MEIOB ( SPATA22 ) in meiosis recombination, which was co-expressed with MEIOB in testis, displayed mutually exclusive expression pattern in samples with LUAD and other cancer types. This reflects the common and unique characteristics of germ and tumour cells. In addition, we found that ncRNAs with testis-specific expression patterns could possibly contribute to carcinogenesis by interacting with these CT genes. These ncRNAs can either promote ( LIN28B and LINC00577 ) or inhibit ( MEIOB and LINC00254 ) nearby genes. We also found that EECTPs may be exclusively activated by mutations in SMGs. In BRCA, this mutually exclusive pattern between PIK3CA and EECTPs achieved statistical significance due to the sufficient sample size. In all cancer types, we found some samples without mutations in SMGs [1] ; therefore, CT genes may serve as complements of mut-drivers. This hypothesis was further strengthened by data from a genomic study on papillary thyroid carcinoma. Our results revealed that demethylation was an important mechanism for the reactivation of CT genes, which was consistent with conventional knowledge of CT gene activation mechanisms [13] , [47] . In conclusion, our study identified hundreds of CT genes in 19 cancer types using publically available databases. We successfully extended the definition of CT antigens to include CT genes (CT proteins and CT-ncRNAs). We used EE patterns to define and identify EECTGs and successfully proved that EECTGs, which might be activated by promoter demethylation or by proximal CT-lncRNAs, could serve as potential sources of epi-drivers in cancer. Generally speaking, these findings expand our knowledge of CT genes and provide new perspectives for identifying epi-driver genes in cancer. Public data sets used in this study We used the multiple public databases involving both normal and tumour tissues to evaluate TSGs and evaluate cancer-specific CT genes and EECTGs. Detailed information of these databases was listed in the Supplementary Table 1 and Supplementary Data 1 . Classification of all genes A total of 50,016 unique genes with expression abundance data (FPKM) from three data sets (GTEx, Illumina Human Bodymap and NJMU-seq) were included in the analysis after integration. ENSEMBL ID (GENCODE v19) was used as an indicator. Genes were classified into the following six categories ( Fig. 1 ) based on specificity measure (SPM) values: (C1) high-confidence testis-specific coding genes: GENCODE-annotated protein-coding genes (v19) with a SPM GTEx >0.9, SPM HBM >0.9 and SPM NJMU >0.9; or b Known CT and SPM GTEx =0, SPM HBM >0.9, SPM NJMU >0.9 and gene copies with identical sequences; (C2) high-confidence testis-specific non-coding genes: GENCODE-annotated non-coding genes (v19) with SPM GTEx >0.9, SPM HBM >0.9 and SPM NJMU >0.9; (C3) moderate-confidence testis-specific coding genes: GENCODE-annotated protein-coding genes (v19) with SPM GTEx >0.9 and either SPM HBM >0.9 or SPM NJMU >0.9; (C4) moderate-confidence testis-specific non-coding genes: GENCODE-annotated non-coding genes (v19) with SPM GTEx >0.9 and either SPM HBM >0.9 or SPM NJMU >0.9; (C5) low-confidence TSGs: genes with SPM GTEx >0.9 but SPM HBM ≤0.9 and SPM NJMU ≤0.9; (C6) non-gene-level TSG: genes with SPM GTEx ≤0.9. To further distinguish genes with testis-specific expression patterns at the transcript level but not at the gene level, we classified G6 into the following two sub-groups using transcript abundance data from GTEx; (C6a) genes with testis-specific transcripts: C6 with SPM GTEx transcript >0.9; (C6b) genes without testis-specific transcripts: C6 with SPM GTEx transcript ≤0.9. Details of SPM value calculations are provided in the Supplementary Information (Methods to evaluate TSGs). To accurately define TSPs, we used expression data curated from gene-specific peptides. We used same SPM criteria to define TSPs ( Supplementary Figure 9 ). Some classical CT genes had similar sequence and shared peptides, such as MAGE family genes, would be missed. To address this issue properly, we used expression profiles at both the protein level and the peptide level and classified all genes into the following four groups: 1 TSPs 2 Testis-specific peptides 3 Proteins that had at least one peptide with testis-specific expression (SPM >0.9). 4 No data: proteins or genes with no protein expression data. 5 Non-TSPs: other proteins. Evaluation of TSGs/ CT genes related to testis-specific regulatory elements Enrichment analysis was applied to evaluate the relationship between TSGs/ CT genes and their nearby testis-specific regulatory elements (TSREs). Four types of TSREs (promoters, methylation levels, ncRNAs and enhancers) were considered. Detailed information concerning the definition and identification of TSREs is listed in the Supplementary Methods . Fisher’s exact test was applied to evaluate the ER, which was calculated as follows: Criteria for cancer-specific CT genes and EECTGs/EECTPs Genes were further grouped as CT genes and EECTGs/EECTPs after considering the above six categories and cancer-related information. CT genes met the following criteria: (1) exhibited testis-specific expression patterns with high confidence (C1); (2) exhibited expression (>5 normalized read counts) in at least 1% of cancer samples. EECTGs met the following criteria: (1) exhibited CT gene expression patterns; (2) exhibited EE ( ) in at least 1% of cancer samples. EECTPs met the following criteria: EECTGs exhibiting testis-specific expression patterns at the protein level. Go analysis was performed using DAVID online tools ( http://david.abcc.ncifcrf.gov/ ). The top 10 enriched clusters were determined by automated functional annotation clustering with default parameters. Evaluation of the relationship between mutations and EECTPs As driver mutations are significantly less frequent than passenger mutations, we used the total mutation number to reflect the burden of passenger mutations. We calculated mutation ratio as follows: The mutation ratio represents the degree of samples driven by mutations for specific genes. The activated number of EECTPs represents the degree of samples driven by EECTPs. Linear regression was used to evaluate the association between the mutation ratio and the activated number of EECTPs. For each SMG, a Wilcoxon’s rank-sum test was used to compare the activated EECTP numbers between mutated and non-mutated samples. Fisher’s exact test was employed to test mutually exclusive patterns between the mutation patterns of SMGs and EE patterns of EECTPs. Relationship between promoter methylation levels and EECTPs The default RnBeads [48] workflow was used for quality control and to preprocess raw idat files produced by the Infinium HumanMethylation450 BeadChip Kit. Beta values for the promoters were extracted from the RnBeads output. Mean beta values were calculated to reflect promoter methylation levels for all EECTPs or for all genes. Linear regression models were applied to evaluate the relationship between promoter methylation and the activated number of EECTPs. For each EECTP, a Wilcoxon’s rank-sum test was used to compare the promoter methylation levels between activated and inactivated samples. DNA copy number analysis and chromosomal instability scarring scoring The global burden of focal CNAs was calculated as the total length of focal copy number (gain and loss) for each individual. The cutoffs for parameter Seg.CN were set to −0.2 and 0.2 to distinguish loss and gain, respectively. Allele-specific copy number analysis was performed with allele-specific copy number analysis of tumours (ASCAT v2.1) (ref. 49 ). Segments of allele-specific copy number profiles were classified into one of the following three non-overlapping types: allele-imbalanced CNAs (AiCNAs), allele-balanced CNAs (AbCNAs) or CnLOH. We calculated the score of each category (S AiCNA , S AbCNA and S CnLOH ) according to methods described previously [38] . S Ai was calculated by summing S AiCNA and S CnLOH , thereby capturing all allelic imbalance events. A Wilcoxon’s rank-sum test was used to compare the global burden of focal CNAs, or S Ai , between the activated and the inactivated samples. In-house mRNA expression data sets We obtained normal human tissue samples ( n =7, 5 normal tissues, Supplementary Data 1 ) to define TSGs. We paired these samples with tumour/adjacent tumour tissues from LUAD patients ( n =24) to validate EECTGs expression patterns. Human tissue samples used for mRNA expression analyses in the NJMU study were collected and handled in accordance with Chinese laws and regulations and were obtained from Affiliated Hospitals of Nanjing Medical University. At recruitment, informed consent was obtained from each subject. Tissues samples were preserved using RNA-later solution. Haematoxylin and eosin-stained sections from each sample were examined by a board-certified pathologist to ensure sampling of representative normal tissue. Total RNA was extracted from tissue samples using the RNeasy Mini Kit (Qiagen, Hilden, Germany) according to the manufacturer’s instructions. The extracted RNA samples were analysed using an Agilent 2100 Bioanalyzer system (Agilent Biotechnologies, Palo Alto, USA) with the RNA 6000 Nano Labchip Kit. Only samples of high-quality RNA (RNA integrity number ⩾ 7.5) were used in the subsequent mRNA sample preparation for sequencing. PolyA-minus RNAs were fractionated from total RNA samples and RNA-Seq libraries were generated by RNA-fragmentation, random hexamer-primed complementary DNA (cDNA) synthesis, linker ligation and PCR amplification using a TruSeq RNA Sample Prep Kit (Illumina, Inc.). The purified DNA libraries were sequenced with an Illumina HiSeq1500 platform (paired-end, 100 base). To maintain consistency with the estimated expression abundance method used for the GTEx and TCGA databases, we estimated the FPKM for normal tissues to evaluate TSGs using the TopHat-Cufflinks protocol (TopHat v2.0.9 and Cufflinks v2.2.1) and normalized read counts (normalized by upper-quantile method) [50] for paired tumour/adjacent tumour tissues to validate EE patterns using the RSEM (RSEM v1.2.12). GENCODE v19 was used as the reference genome. The RNA-Seq data have been deposited at ArrayExpress (E-MTAB-4063). Cell culture Human lung cancer cell line A549 was cultured in RPMI 1640 (Gibco) supplemented with 10% FBS. Cells were maintained at 37 °C with 5% CO 2 . The sources of the cell line and mycoplasma contamination were evaluated by Beijing JianLian Gene Technology Co., Ltd, on September 2013. DNA prepared from our A549 cells using a commercial Chelex100 kit was analysed by STR (Short tandem repeat) profiling. Our A549 cell line is considered to be ‘identical’ to a culture in the ATCC A549 STR database; the entered STR profile yields a 100% match (11 of 11 loci) to the result set. No cross-contaminated cell lines or mycoplasma contamination was detected. Lentiviral infection was performed as follows: HEK-293T cells were co-transfected with pHelper 1.0 and pHelper 2.0 constructs and packaging plasmids. The progeny viruses released from HEK-293T cells were filtered, collected with a centrifugal filter unit (Centricon Plus-20, P31925, Millipore) and used to infect A549 cells. The lentivirus infected these two cancer cells via 8 mg ml −1 Polybrene mixed in RPMI 1640. RNA isolation and quantitative real time-PCR Total RNA was extracted using TRIzol Reagent (Invitrogen) and reverse transcribed using the High Capacity RNA-to-cDNA Kit (Takara). cDNA was quantified using TaqMan Gene Expression Master Mix through an ABI 7900HT System (Applied Biosystems; Expression TaqMan lot number: MEIOB -1119967; LINC00254 -1175109). Protein isolation and western blotting Cells were lysed in mammalian protein extraction reagent (Beyotime). After quantification using a BCA protein assay kit (Beyotime), total proteins were separated by SDS–PAGE under denaturing conditions and transferred to PVDF membranes (Millipore). Membranes were blocked in 5% non-fat milk and incubated with and anti-MEIOB (ab150886, respectively; Abcam), followed by incubation with anti-rabbit secondary antibodies. We used seeBlue@ Plus 2 Prestained (lot#:1368753) as indicators of proteins. Immunoreactive proteins were visualized using a molecular imager (Bio-Rad). Uncropped scans of western blots were included in the Supplementary Fig. 8d . Gene deletion Guide RNAs were designed to recognize chr16:1911998–1912070 ( MEIOB ) and chr16:1928364–1934279 ( LINC00254 ) (hg19) and cloned into PGL3. Constructs were introduced into lung cancer cell lines (A549) using Lipofectamine 2000 reagent (Invitrogen) along with a plasmid encoding Cas9. Cells were sorted using a flow cytometer to capture cells with high green fluorescent protein signals. Colonies were grown from single cells. Complete deletion of both lncRNA alleles was confirmed by PCR using primers flanking lncRNA. The deletion of these two genes was confirmed by both sequencing and western blotting. Single guide RNA (sgRNA) sequences and primers used for amplifying the sgRNA target site and for sequencing are listed in Supplementary Table 2 . Cell proliferation assay Treated cells were seeded in 96-well plate and the viability of cells was measured with a Cell Counting Kit-8 (CCK8, Dojindo, Japan) daily for 5 days. Briefly, 10 μl of CCK8 solution was added to each well with 100 μl RPMI 1640 and incubated at 37 °C for 2 h. The absorbance was measured at wavelengths of 450 nm. We also used an 5-ethynyl-2’-deoxyuridine (EdU) array to confirm the cell viability between differently treated cells. According to the manual of a EdU labelling/detection kit (Ribobio, Guangzhou, China), 50 M EdU labelling medium was added to the cell culture to allow incubation for 2 h at 37 °C under 5% CO 2 . Subsequently, cultured cells were fixed with 4% paraformaldehyde (pH 7.4) for 30 min and incubated with glycine for 5 min. After washing with PBS, staining with anti-EdU working solution was performed at room temperature for 30 min. Following washing with 0.5% TritonX-100 in PBS, the cells were incubated with 5 g ml −1 Hoechst 33342 dye at room temperature for 30 min, followed by observation under a confocal laser scanning microscope (ECLIPSE-Ti, Nikon). The percentage of EdU-positive cells was calculated from nine random fields in three wells. The results are given as mean±s.d. of cell number relative to the vehicle control. Colony formation assay Cells were cultured in six-well plates (300 cells per well) for 3 weeks and then fixed with methanol for 20 min at room temperature. After fixation, colonies were stained with 0.5% crystal violet for 30 min. Images of all wells were captured at room temperature and were counted by hand with the aid of imaging software. The results are given as mean±s.d. of cell colonies relative to the vehicle control. Migration and invasion Cell migration and invasion were studied using Costar Transwell plates (6.5 mm diameter insert, 8.0 mm pore size, polycarbonate membrane; Corning Sparks, MD). Lung cancer cells were plated at a density of 2 × 10 4 cells per 200 μl in the Transwells 1 day for migration and 2 days for invasion before the migration experiment. The cells were then fixed with methanol for 20 min at room temperature. After fixation, colonies were stained with 0.5% crystal violet for 30 min. The membranes were then dried, inverted and mounted on microscope slides for analysis. Images of four random fields for each membrane were captured at room temperature via a Nikon microscope and were counted by hand with the aid of imaging software. Counts from all 10 fields were averaged to obtain a mean cell count for each membrane. All experiments were performed at least three times with n =3 per trial. The results are given as mean±s.d. of cell migration and invasion relative to the vehicle control. Cell cycle The cell cycle was analysed by flow cytometry. For cell cycle analysis, transfected lung cancer cells were suspended in 75% ethanol overnight and centrifuged at 1,000 r.p.m. Following two washes of the cell pellets in PBS, 50 mg ml −1 propidium iodide (PI) and 100 g ml −1 DNase-free RNase A was added and the cell pellet was re-suspended. Following incubation for 30 min at 37 °C, the samples were analysed by flow cytometry. Cell cycle distribution was further analysed with Cell Quest software (Becton Dickinson, San Jose, CA) and Mod Fit LT (Verity Software House, Topsham, ME). Accession codes: The RNA-Seq data have been deposited in the ArrayExpress database under accession code E-MTAB-4063. How to cite this article: Wang, C. et al . Systematic identification of genes with a cancer-testis expression pattern in 19 cancer types. Nat. Commun. 7:10499 doi: 10.1038/ncomms10499 (2016).